Concentration and chemical-state profiles at heterogeneous interfaces with sub-nm accuracy from standing-wave ambient-pressure photoemission Heterogeneous processes at solid/gas, liquid/gas and solid/liquid interfaces are ubiquitous in modern devices and technologies but often difficult to study quantitatively. Full characterization requires measuring the depth profiles of chemical composition and state with enhanced sensitivity to narrow interfacial regions of a few to several nm in extent over those originating from the bulk phases on either side of the interface. We show for a model system of NaOH and CsOH in an ~1-nm thick hydrated layer on α-Fe 2 O 3 (haematite) that combining ambient-pressure X-ray photoelectron spectroscopy and standing-wave photoemission spectroscopy provides the spatial arrangement of the bulk and interface chemical species, as well as local potential energy variations, along the direction perpendicular to the interface with sub-nm accuracy. Standing-wave ambient-pressure photoemission spectroscopy is thus a very promising technique for measuring such important interfaces, with relevance to energy research, heterogeneous catalysis, electrochemistry, and atmospheric and environmental science. Solid/gas, liquid/gas and solid/liquid interfaces play a major role in many important areas of science and technology, for example, in energy generation, electrochemistry, corrosion, environmental science and information technology, yet pose experimental challenges for the investigation of their chemical and structural properties on the molecular scale. For example, the electrical double layer has been studied for over 100 years, and yet is not fully understood [1] , [2] . Characterizing such interfaces requires enhancing the signal from the narrow interfacial regions over those originating from the layers on either side of them. Ambient-pressure X-ray photoelectron spectroscopy (APXPS, APPS), in which the pressure near the sample is maintained in the multi-Torr regime, is a rapidly growing technique that permits studying surface chemical interactions in more realistic conditions compared with previous studies at or near ultrahigh vacuum [3] , [4] , [5] , [6] , [7] , [8] . APXPS has been applied to a wide range of interfaces, including recently solid–liquid interactions in an electrochemical cell in operando [9] , [10] . However, APXPS still cannot quantitatively investigate interfaces in an element- and chemical-state-specific way with sub-nanometre (nm) resolution, especially for more deeply buried interfaces, such as those in a solid–liquid system. Probing depths in APXPS are controlled by photoelectron inelastic mean free paths (IMFPs), which are, for typical kinetic energies of a few hundred to a thousand eV, a maximum of a few tens of Angstroms [11] . Varying the photon energy so as to change the IMFP is one way of providing depth resolution in APXPS [7] , but the data analysis involves a convolution integral that may need additional compositional constraints to be solved uniquely [12] . Tailoring the exciting X-ray wave field into a standing wave is a method for achieving greater depth sensitivity in photoemission, and it has been applied to a number of solid/solid interfaces [13] , [14] , [15] , [16] , [17] . In fact this method has also been applied previously in X-ray reflectivity and emission measurements on multilayer systems and at the solid–liquid interface [2] , [18] , but photoemission has the significant advantages of being more interface sensitive due to the shorter escape depths of electrons and of providing more direct chemical-state information from chemical shifts in core-level binding energies. We here combine standing-wave and ambient-pressure photoemission (SWAPPS) to study the regions near a solid/liquid and a liquid/gas interface, represented by a hydrated, mixed NaOH/CsOH layer on a polycrystalline haematite surface. We show that SWAPPS can determine the chemical-state resolved depth profiles of every element in the sample with sub-nm resolution. For example, we show that the Na and Cs ion have distinctly different depth distributions. This work thus demonstrates the high future potential of SWAPPS for studying a broad range of interface phenomena. The sample The sample configuration is shown in Fig. 1a . As discussed further in Methods, a strong standing wave (SW) was created in the sample by growing a haematite layer on a synthetic multilayer mirror for X-rays, which consists of a number of bilayers of low-Z/high-Z material (here Si/Mo), and then scanning the incidence angle over the first-order Bragg’s reflection of the mirror. This scan sweeps the SW vertically through the sample over roughly one-half of its period, and generates what is termed a rocking curve (RC) of various individual core-level photoelectron peak intensities. We present below experimental results together with theoretical photoemission calculations that quantitatively incorporate the standing-wave field [19] , [20] . Comparison of the experimental RCs immediately provides some qualitative information as to relative depths of all components of the interface and adjacent bulk regions, with the theoretical calculations finally providing a quantitative model of depth distributions for all of the chemical components present, with sub-nm accuracy. 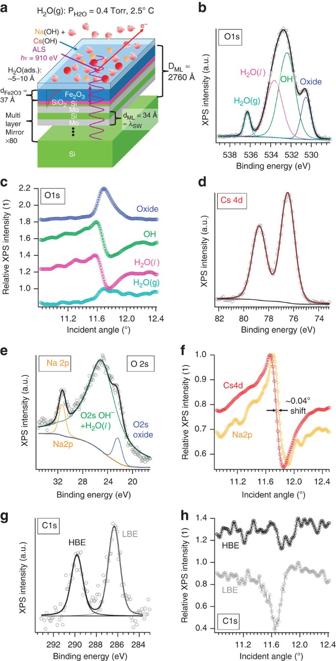Figure 1: The sample configuration, together with some key rocking curves for the various elements in the sample. (a) The sample configuration, with some relevant dimensions noted. (b) An O 1s spectrum, resolved into four components by peak fitting. The component labelled OH−may also contain contributions from carboxyl and bicarbonate species. (c) The rocking curves derived from the four components of (b). (d) A Cs 4d spectrum, including peak fitting. (e) Analogous overlapping Na 2p and O 2s spectra, with peak fitting. (f) The rocking curves for Cs 4d and Na 2p derived from spectra such as those in (d) and (e). (g) A typical C 1s spectrum, showing the two components, one at low binding energy (LBE) and one at higher binding energy (HBE). (h) The rocking curves for the two C 1s components. Figure 1: The sample configuration, together with some key rocking curves for the various elements in the sample. ( a ) The sample configuration, with some relevant dimensions noted. ( b ) An O 1s spectrum, resolved into four components by peak fitting. The component labelled OH − may also contain contributions from carboxyl and bicarbonate species. ( c ) The rocking curves derived from the four components of ( b ). ( d ) A Cs 4d spectrum, including peak fitting. ( e ) Analogous overlapping Na 2p and O 2s spectra, with peak fitting. ( f ) The rocking curves for Cs 4d and Na 2p derived from spectra such as those in ( d ) and ( e ). ( g ) A typical C 1s spectrum, showing the two components, one at low binding energy (LBE) and one at higher binding energy (HBE). ( h ) The rocking curves for the two C 1s components. Full size image Rocking curves In Fig. 1b a typical O 1s spectrum is shown, with four distinct peaks resolved, which are due to water in the gas phase above the sample, liquid-like water adsorbed on and above the Fe 2 O 3 surface, oxygen in the alkali hydroxides and possibly also in carboxyl- or carbonate species that we cannot resolve in this peak and that we designate simply as OH − and oxide oxygen from the Fe 2 O 3 . The assignment of these peaks is based on previous APXPS studies [21] . Gas-phase peaks are seen in all APXPS spectra, as the X-ray beam is wide enough to pass through the gas above the sample in a region also seen by the spectrometer [6] , [7] . The distinction of the peaks from H 2 O( ℓ ) and OH − is further justified by examining their different relative intensities through the rocking curve scan (results not shown here). From an analysis of experimental relative core peak intensities using the SESSA XPS simulation program [22] , [23] the adsorbed water layer is found to be about 5–10 Å thick, although we will later see that the analysis of the SWAPPS results provides a much more accurate value for this thickness of ~10 Å. This thickness is significantly larger than that of H 2 O on pure metal oxide surfaces at our relative humidity of ~8% (refs 21 , 24 ). This is due to facilitation of water adsorption by Cs + , Na + and OH − ions and formation of their solvation shells. Figure 1c shows O 1s RC data, based on spectral deconvolution by peak fitting as shown in 1(b). All four peaks exhibit the effects of the SW scanning through the adsorbed layer, with relative magnitudes as high as 50%, including even the gas-phase water, which is modulated due to the changes in reflectivity that influence the total E-field strength above the sample. All RCs are normalized to have a maximum value of 1.0, with vertical shifts to permit overlapping them, so the fractional changes can easily be discerned from the abscissa scale. The distinct shapes of the different O 1s RCs directly indicate that the chemical species associated with the respective photoemission peak have different average vertical positions in the sample. The O 1s(OH − ) and O 1s(H 2 O) RCs do not show a significant shift, but nonetheless exhibit slightly different behaviour in the wings of the curves, with O 1s(H 2 O) being more intense, suggesting not quite identical depth distributions, and we explore this further below. Figure 1d shows the Cs 4d spectrum whose peak-fit intensity was used to derive the RC in Fig. 1f . Figure 1e shows the overlapping Na 2p and O 2s valence spectra from which the Na 2p RC in Fig. 1f was derived. From Fig. 1f , we find a small but reliable shift of 0.04° between the Cs 4d and Na 2p RCs in the steeply sloping regions of the two curves near the Bragg’s angle of the multilayer, as well as different shapes in the wings away from these regions, with Cs having higher intensity both below and above the Bragg’s angle. Thus, the data alone suggest different depth distributions of Cs + and Na + . The C 1s photoelectron spectrum contains two components ( Fig. 1g ), which follow distinctively different RC behaviour ( Fig. 1h ). The low binding energy (LBE) component, which we tentatively assign to hydrocarbon-like C, exhibits the largest fractional SW modulation, which is typically a sign of a thinner layer, with thicker layers averaging over the phase of the SW and thus reducing the intensity modulation in a RC. The modulation of the high binding energy (HBE) component, probably reflecting the presence of carboxylic and/or bicarbonate groups, shows a much smaller amplitude, and this in turn suggests a much broader depth profile for this species that thus averages over the phase of the SW. The presence of carbon in different oxidation states in the adsorbed layer on our sample under in situ measurement conditions at this high a relative humidity is due to both the sample preparation protocol as well as the inherent background contamination in experiments at elevated pressures, and has been observed in a number of experiments under similar conditions [21] . Depth sensitivity estimate To provide some first-order semi-quantitative insight into the depth resolution of these RC measurements, Fig. 2 shows model calculations of the shapes of rocking curves for emission from a water ‘delta layer’ of 1 Å thickness that was successively moved through a 10 Å water layer, calculated at the average O 1s kinetic energy, but which could also represent Cs + , Na + or other species, as a function of distance Δz above the Fe 2 O 3 surface. 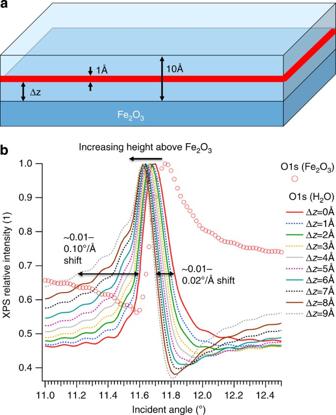Figure 2: A set of model calculations for assessing the sensitivity of SWAPPS rocking curves to depth. (a) The model sample geometry used for scanning a water ‘delta layer’ of 1 Å thickness through a water film of 10 Å thickness on top of Fe2O3to assess the change in rocking curves. (b) A summary of calculated rocking curves for O1s from the delta layer, with steps in heightΔzof 1 Å. A reference rocking curve for O 1s emission from Fe2O3is also shown. The typical changes seen to the right and to the left of the curves are also indicated. Figure 2a illustrates the model geometry on top of the nominal structure of the mirror. These calculations have been carried out using a versatile X-ray optics program described elsewhere that has been used in a number of previous SW photoemission studies of multilayer solid systems [20] . The results of these calculations in Fig. 2b indicate that a 0.04° shift at the maximum slope region can be associated with a 4 Å difference in position, but more so that the behaviour in the wings of the rocking curve is also sensitive to the vertical position, showing even larger changes in angular width on the low-angle side of the rocking curve. Thus, we can further suggest that Cs + is on average a few Å farther from the Fe 2 O 3 surface, and by the absence of subsidiary Kiessig interference fringes that are somewhat more clearly visible for Na + , that its distribution is probably broader. A more detailed analysis incorporating some assumed distributions in depth for both Cs + and Na + is necessary to be fully quantitative. This quantitative analysis of our data is described in the following. Figure 2: A set of model calculations for assessing the sensitivity of SWAPPS rocking curves to depth. ( a ) The model sample geometry used for scanning a water ‘delta layer’ of 1 Å thickness through a water film of 10 Å thickness on top of Fe 2 O 3 to assess the change in rocking curves. ( b ) A summary of calculated rocking curves for O1s from the delta layer, with steps in height Δz of 1 Å. A reference rocking curve for O 1s emission from Fe 2 O 3 is also shown. The typical changes seen to the right and to the left of the curves are also indicated. Full size image Quantitative analysis The optimization of the structure was done by first carrying out calculations of the Fe 3p (oxide), O 1s(oxide), summed [O 1s(OH − )+O 1s(H 2 O(l)] RCs, and the C 1s LBE RC, and treating as fitting parameters the vertical positions and thicknesses of the Fe 2 O 3 layer, the liquid-like H 2 O+OH − layer and the layer containing LBE C contaminants, together with the thicknesses of the mutual interdiffusion between these three layers, which were assumed to be linear in form. Self-consistency requires that Fe 3p(oxide) and O 1s(oxide) be associated with the same depth distribution for Fe 2 O 3 , thus increasing the final accuracy of the structure determination for these layers. At each step, the goodness-of-fit of theoretical predictions generated by the code was judged by a χ 2 sum, divided by the number of data points. A modified fast-converging Newton method with successive over-relaxation was used to find optimum parameters [25] . 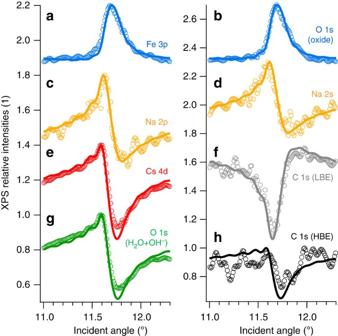Figure 3: A comparison of the experimental rocking curves for various core-level intensities with theoretical calculations based on the optimized sample configuration defined inFig. 4. (a) Fe 3p, (b) O 1s (oxide), (c) Na 2p, (d) Na 2s, (e) Cs 4d, (f) low binding energy C 1s, (g) O 1s (OH−+H2O) (h) high binding energy C 1s. Figure 3a,b,f and g compares experiment and theory from this step, and Fig. 4a presents the resulting depth distribution. In the following step, the same technique was used to fit the Cs 4d and Na 2p RCs, and derive their depth distributions. Self-consistency again could be used in requiring that Na 2s (not shown) and Na 2p be associated with the same distribution for Na + . The results from this second step are further shown in Fig. 3c–e , and summarized separately in Fig. 4b, c . As a final step, the HBE C rocking curve was fit, with results shown in Fig. 3h , and its much broader distribution given in Fig. 4d , which summarizes all of the depth distributions in the form of curves. Excellent agreement is found between experiment and X-ray optical theory for all of the core-level rocking curves, and our estimated accuracy in deriving these structural parameters is ±1-2 Å. Figure 3: A comparison of the experimental rocking curves for various core-level intensities with theoretical calculations based on the optimized sample configuration defined in Fig. 4 . ( a ) Fe 3p, ( b ) O 1s (oxide), ( c ) Na 2p, ( d ) Na 2s, ( e ) Cs 4d, ( f ) low binding energy C 1s, ( g ) O 1s (OH − +H 2 O) ( h ) high binding energy C 1s. 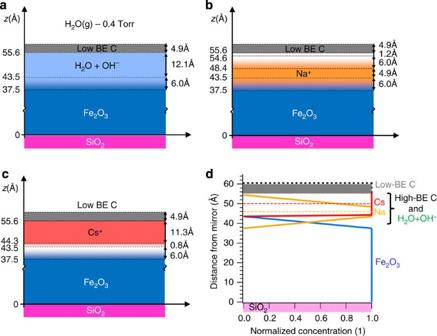Figure 4: The final depth distributions in the sample as derived by fitting experimental rocking curves to theory. Depth distributions for (a) Fe2O3, the OH−+H2O electrolyte layer treated as a unit, and the low binding energy C, (b) the Na+layer and (c) the Cs+layer. In (d), the concentration distributions of all species are shown overplotted as curves, with the horizontal scale in normalized atomic concentrations that are unity at the maximum for each species. Full size image Figure 4: The final depth distributions in the sample as derived by fitting experimental rocking curves to theory. Depth distributions for ( a ) Fe 2 O 3 , the OH − +H 2 O electrolyte layer treated as a unit, and the low binding energy C, ( b ) the Na + layer and ( c ) the Cs + layer. In ( d ), the concentration distributions of all species are shown overplotted as curves, with the horizontal scale in normalized atomic concentrations that are unity at the maximum for each species. Full size image Figure 4 further permits concluding that the Fe 2 O 3 surface has an effective roughness and/or interface interdiffusion distance of about 6 Å. In fact, atomic force microscopy measurements on the Fe 2 O 3 surface after measurement and after cleaning with distilled water showed a root mean squared roughness very close to this value. Figure 4 also shows that the Na + ions are located at an average distance of 5.5 Å above the mean of the Fe 2 O 3 surface and extend over about 11 Å in depth, while the Cs + ions are located at a larger average distance of 9.5 Å above the mean Fe 2 O 3 surface and extend over about 12 Å in depth. Cs + is on average 4 Å further from the surface than Na + , in qualitative agreement with our discussion of the model rocking curve simulations presented in Fig. 2b . The LBE C-containing contaminants are localized within a thin layer of about 5 Å thickness at the liquid/gas interface and thus appear to be hydrophobic, while the HBE C-containing contaminants, possibly carboxyl or bicarbonate species, are spread over the whole-depth range of the ‘wet’ layer without a significant concentration gradient. Through separate fitting of the O 1s OH − and O 1s H 2 O RCs (not shown here), the OH- ions and the water molecules are found to be virtually identical in depth distribution, with OH − being deeper in its distribution by ~1 Å, although this is at the limit of our resolution and would require data of higher statistical accuracy to resolve more quantitatively. At this point, we thus conclude that OH − and H 2 O have very nearly the same depth distribution. Quantitative concentrations In the usual sense of XPS quantitative analysis, we can also make use of the relative core peak intensities to estimate the true concentrations of several important species in cm −3 . This was done by comparing the relative intensities of all of the peaks shown in Fig. 3a–e , as measured off the Bragg reflection to yield a uniform X-ray flux throughout the sample, with calculated relative intensities from the SESSA XPS simulation program [22] , [23] . The relevant concentrations in the layer structure of Fig. 4 were varied in the calculations to give the best agreement between experiment and theory. The Fe 3p and O 1s(oxide) intensities provide internal references for the concentration of the Fe and O atoms in Fe 2 O 3 (3.95 × 10 22 cm −3 for Fe and 5.93 × 10 22 cm −3 for O). The IMFPs were assumed to be 18 Å for Fe 3p and 10 Å for O 1s in Fe 2 O 3 , and to be 37 Å for the complex overlayers, which are predominantly OH − (including as before what might be carboxylic or bicarbonate species)+H 2 O, with these IMFP numbers derived from a combination of the Tanuma-Powell-Penn formula [11] and theoretical and experimental results for H 2 O [26] . The final results of these calculations yield concentrations in the ‘bulk’ central regions of each layer of Cs + and Na + are 1.36 × 10 22 cm −3 and 0.64 × 10 22 cm −3 , respectively. As a final result, the effective concentration of the ‘solution’ in this thin aqueous layer is thus very high at ~[Cs + +Na + ]≈22 M+10 M=32 M. Carrying this calculation one step further, we estimate about two monolayers total of Cs and one monolayer total of Na in the adsorbed layer on Fe 2 O 3 . The fact that the Cs + and Na + concentrations are not equal is easily explained by differing degrees of hydration of the solid CsOH and NaOH that were weighed in making up the initial solutions. The concentrations of other species based on O 1s and C 1s spectra could not be determined accurately due to a lack of knowledge of the spectrometer transmission as a function of kinetic energy, but could be in future studies using the SWAPPS method with proper calibration. Depth-dependent binding energies As a final aspect of our data, we show in Fig. 5 binding energy changes with depth that can be observed as the SW is scanned through the sample. In Fig. 5a is plotted the variation of the electric field intensity with depth and incident angle, with the profiles of the different chemical species indicated on top of it. The positions of the SW maxima are obvious from the bright roughly elliptical spots, and the scanning in vertical position is obvious from the slopes of the main axis of these spots. The blue arrows indicate extrema in the SW depth from nearer to the Fe 2 O 3 surface to nearer to the top surface of the sample. 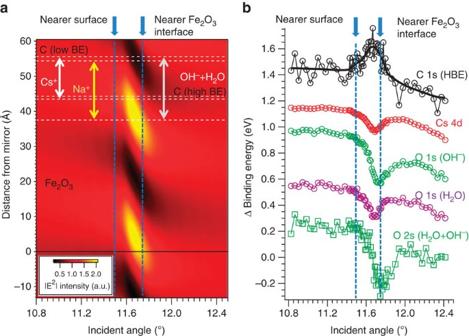Figure 5: Comparison of calculated standing-wave electric field depth profiles as a function of X-ray incidence angle to core-level binding energies also as a function of incidence angle. (a) The calculated standing-wave profile of electric field intensity (|E2|) as a function of depth and incident angle. The two arrows and dashed lines indicate locations at which the field will focus more on the Fe2O3interface or more towards to the top surface of the sample. (b) The variation in binding energy for some selected core-level peaks as incidence angle is scanned through a rocking curve. The curves are all on the same relative scale, but have been offset for visibility. These changes are different in position and sign, thus indicating that they cannot be due to sample charging or purely instrumental effects. Figure 5b now shows the binding energy of several core levels as an RC is scanned, and it is clear that, as the SW moves through the sample, there are significant shifts of 0.2–0.4 eV. The general downward slope in these curves is a purely instrumental effect that is found in all binding energies. The fact that all of these binding energy curves show different positions and shapes, although with OH − and H 2 O being very similar to one another, and that they are not all of the same sign, argues strongly that these are due to bonding or local potential changes with depth in the sample. A detailed analysis of these shifts would require theoretical calculations beyond the scope of this paper, but these results thus point out an additional strength of the SWAPPS method, being able to study chemical states or electrostatic potentials in a depth-resolved way near an interface. Figure 5: Comparison of calculated standing-wave electric field depth profiles as a function of X-ray incidence angle to core-level binding energies also as a function of incidence angle. ( a ) The calculated standing-wave profile of electric field intensity (|E 2 |) as a function of depth and incident angle. The two arrows and dashed lines indicate locations at which the field will focus more on the Fe 2 O 3 interface or more towards to the top surface of the sample. ( b ) The variation in binding energy for some selected core-level peaks as incidence angle is scanned through a rocking curve. The curves are all on the same relative scale, but have been offset for visibility. These changes are different in position and sign, thus indicating that they cannot be due to sample charging or purely instrumental effects. Full size image We now comment on the relationship of our results to what is known about the adsorption of alkali ions on haematite and other oxides. Previous studies have demonstrated preferential adsorption of Na + over Cs + ions on haematite and other metal oxide surfaces [27] , [28] , [29] , [30] , [31] . The ionic adsorption sequence: Li + >Na + >K + >Cs + , known as the inverse lyotropic adsorption sequence, was first observed for rutile TiO 2 by Bérubé et al . based on indirect capacity measurements [27] and later confirmed for various other metal oxides, including Al 2 O 3 (ref. 29 ) and Fe 2 O 3 (refs 30 , 31 ). The sequence has been explained on the basis of the ionic double-layer model, often referred to as the ‘structure-making–structure-breaking’ model. According to this picture, the adsorption of inorganic ions on the surface of a metal oxide in contact with an aqueous liquid phase is governed by the extent to which the surface and the ions disrupt or promote the structural order of water at the surface. Ions that cause a similar effect on the water structure as the surface tend to be easily adsorbed, while ions that affect the water structure differently from the surface tend to be excluded. Thus, when the surface is characterized by a strong affinity for water, then small, heavily hydrated ions, such as Li + and Na + , which do not significantly affect the water structure in the surface region, are preferentially adsorbed over larger, less hydrated ions, such as K + and Cs [27] , [31] . Haematite, along with Al 2 O 3 , TiO 2 and ZnO, belongs to this class of ‘structure promoting’ materials, exhibiting preferential adsorption of Na + over Cs + . The opposite is the case for ‘structure breaking’ materials, such as SiO 2 , V 2 O 5 and WO 3 , which exhibit preferential adsorption for larger ions such as Cs + rather than small ones such as Li + and Na + (ref. 28 ). Dumont et al . [28] have in fact shown that the ‘structure promoting’ or ‘structure breaking’ properties of a surface can be predicted based on the heat immersion value, or equivalently the point of zero charge (pzc) of the material, with pzc=4 roughly being the value separating the two classes of compounds. Our study thus confirms the preferential adsorption of Na + over Cs + on Fe 2 O 3 , providing for the first time a direct probe of the distribution of different chemically distinct species through a solid/liquid interface, including the detection of their chemical states and potential evolution near the interface. We conclude that the Cs + ions are practically excluded from the Fe 2 O 3 surface, populating predominantly the outer atomic layers closer to the liquid/gas interface. The intrinsic roughness of the Fe 2 O 3 surface affects mostly the Na + -containing layer and less so the Cs + and LBE C-containing layers, which have sharper interfaces. This might indicate that the outer layers are predominantly influenced by the properties of the liquid/gas interface, with the roughness of the solid surface partly ‘screened’ by the inner Na + layers. SWAPPS thus provides quantitative information on the thickness of the various layers and the roughness of each interface. We have thus demonstrated that combining ambient-pressure photoemission and standing-wave photoemission can yield depth profiles of chemical species and chemical states in a liquid-like environment above a solid surface with unprecedented detail. For the specific study case of Fe 2 O 3 haematite in contact with an aqueous NaOH/CsOH electrolyte, the spatial distributions of the electrolyte ions and the carbon contaminants across the solid/liquid and liquid/gas interfaces were directly probed. Absolute concentrations of species were determined. Binding energy shifts with depth were observed that provide additional information on the detailed bonding and/or depth-dependent potentials in the system. We have thus obtained quantitative insight into the roughness and microscopic nature of the interfaces and the atomic layers forming between them, demonstrating significant spatial separation of the Na + and Cs + ions, as well as of the different carbon species. The results for Na + and Cs + are furthermore consistent with previous studies of the relative adsorption strengths of these ions on metal oxide surfaces. Although the technique requires growing the sample on some kind of multilayer mirror, there are many possible material choices for this [32] , and the sample layers involved are often polycrystalline or amorphous and so often simple to grow on such mirrors, so we do not view sample synthesis as a major limitation for future applications. A very well-defined beam of at most ~0.01 degrees in angular divergence is also required, which probably requires using synchrotron radiation or free-electron lasers sources, but many APXPS facilities at such sources are available by now. Depending on the photon energy, interfaces below covering layers of a few nm (soft X-rays up to ~1 keV) or of a few 10 s of nm (~5–10 keV) should be capable of study. Carrying out such SWAPPS measurements with harder X-ray excitation in the multi-keV regime should also permit looking through relatively thick liquid electrolyte films with in operando condition [9] , [10] , thus providing a truly quantitative picture of the solid/liquid interface and the electrochemical double layer for the first time. Ambient pressures that may go up to 1 atm should also be possible, in particular with hard X-ray excitation. Future time-resolved SWAPPS studies using free-electron laser [33] or high-harmonic generation light sources [34] would also permit, via pump-probe methods, looking at the timescales of processes at interfaces on the femtosecond timescale. Finally, doing photoelectron microscopy (PEEM) has already been demonstrated in APXPS [35] and separately with SW excitation for enhanced depth resolution [36] , so future SWAPPS-PEEM studies should provide a true three-dimensional picture of complex interfaces. The range of future applications and measurement scenarios for SWAPPS is thus enormous. Sample preparation We have obtained our SWAPPS data for the different layers and interfaces of hydrated NaOH and CsOH on the surface of a thin film of α-Fe 2 O 3 , which was grown on a Si/Mo multilayer mirror. Figure 1a shows the sample configuration. The Si/Mo mirror was grown at the Lawrence Berkeley National Laboratory (LBNL) Center for X-Ray Optics. The multilayer mirror consisted of 80 repeats of a Si-15 Å/Mo-19 Å bilayer, yielding a repeat distance of d ML =34 Å that can also be shown to be very close to the SW period λ SW at the Bragg reflection angle [13] . A layer of Fe 2 O 3 of nominal 37 Å thickness was grown on top of this mirror in the Liu Laboratory at UC Davis by reactive magnetron sputtering in an ultrahigh vacuum chamber with a base pressure of 9 × 10 −9 torr. X-ray diffraction showed the layer to be either amorphous or nanocrystalline, and Fe 2p core X-ray photoemission, Fe L-edge X-ray absorption and magnetometry confirmed it to be α-Fe 2 O 3 haematite. CsOH and NaOH were chosen as the electrolytes for two reasons: they are much different in size, and so might be expected to show different depth distributions. OH − anions are also expected to be less prone to beam damage than, for example, halides [37] , due to the presence of water vapour. The CsOH/NaOH layer was prepared by depositing a droplet of 0.01 M CsOH/0.01 M NaOH solution onto the sample. The bulk of the solution was then blown away by dry N 2 , leaving a few monolayers of CsOH+NaOH on the Fe 2 O 3 surface. The surface was then rehydrated inside the measurement chamber by exposing it to 0.4 Torr water vapour at a temperature of 2.5 °C, resulting in a relative humidity of ~8% with respect to the sample. Na + and Cs + were chosen as cations for their identical charge and different ionic radii. The influence of beam damage was checked in our experiments and found to be negligible. Photoemission experiments The photoemission measurements were carried out at the LBNL Advanced Light Source, using the ambient-pressure photoemission system at the Molecular Environmental Science beamline 11.0.2 (ref. 38 ). The SWAPPS measurements were carried out using a photon energy of 910 eV, corresponding to an X-ray wavelength of λ x =13.6 Å. With d ML equal to the mirror bilayer spacing, this yields a first-order Bragg angle of arcsin[λ x /2 d ML ]=11.6°, about which the incidence angle was scanned to yield RCs for core levels of every element in the sample. For reference, the IMFP of Fe 3p electrons emitted from Fe 2 O 3 at this photon energy is estimated to be 18 Å; thus, we see through the Fe 2 O 3 layer to some degree and signal is also detected from the Si and Mo on which the sample was grown. We also expect to see weaker Kiessig fringe features due to reflection from the top and bottom of the sample adjacent to the Bragg effects. These have oscillations given by arcsin[mλ x /2 D ML ], where m is the order and D ML is the total thickness of the sample, in this case ~80 × 34+37≈2,760 Å. A simple calculation [13] indicates these fringes are separated by about 0.14°, with these fringes in fact being observed in theoretical calculations, and to some degree also in experiment. How to cite this article : Nemšák, S. et al . Concentration and chemical-state profiles at heterogeneous interfaces with sub-nm accuracy from standing-wave ambient-pressure photoemission. Nat. Commun. 5:5441 doi: 10.1038/ncomms6441 (2014).